In-line alignment and Mg2+coordination at the cleavage site of theenv22twister ribozyme Small self-cleaving nucleolytic ribozymes contain catalytic domains that accelerate site-specific cleavage/ligation of phosphodiester backbones. We report on the 2.9-Å crystal structure of the env22 twister ribozyme, which adopts a compact tertiary fold stabilized by co-helical stacking, double-pseudoknot formation and long-range pairing interactions. The U-A cleavage site adopts a splayed-apart conformation with the modelled 2′-O of U positioned for in-line attack on the adjacent to-be-cleaved P-O5′ bond. Both an invariant guanosine and a Mg 2+ are directly coordinated to the non-bridging phosphate oxygens at the U-A cleavage step, with the former positioned to contribute to catalysis and the latter to structural integrity. The impact of key mutations on cleavage activity identified an invariant guanosine that contributes to catalysis. Our structure of the in-line aligned env22 twister ribozyme is compared with two recently reported twister ribozymes structures, which adopt similar global folds, but differ in conformational features around the cleavage site. The discovery and structural characterization of group I [1] , [2] and group II [3] , [4] , [5] introns have provided unique mechanistic insights into divalent cation-catalysed phosphodiester bond cleavage reactions. By contrast, structure-function studies on small self-cleaving ribozymes that promote rate-enhanced site-specific phosphodiester bond cleavage, have identified alternate catalytic strategies whereby predominantly nucleobase-specific acid–base catalysis mediates cleavage chemistry [6] , [7] . Thus, although the hepatitis delta virus ribozyme [8] , [9] , [10] , [11] does employ a divalent cation in the active site for catalysis, the remaining small self-cleaving ribozymes including hammerhead [12] , [13] , [14] , hairpin [15] , [16] , [17] , [18] , glmS [19] , [20] , [21] , hepatitis delta [10] , [22] , [23] , [24] and Varkud Satellite [25] employ principles of general acid–base and electrostatics for catalysis. These small self-cleaving ribozymes are widely distributed in nature [26] and are essential for rolling-circle-based replication of satellite RNAs [12] , [15] . They facilitate phosphodiester bond-cleavage (and re-ligation) reactions occurring through an S N 2-based mechanism, where the activated 2′-OH of the preceding nucleotide is positioned for in-line attack on the to-be-cleaved P-O phosphodiester bond, resulting in the formation of 2′,3′-cyclic phosphate and 5′-OH groups. The role of geometric constraints, nucleophile activation, stabilization of the transition state and protonation of the leaving group as contributors to small self-cleaving ribozyme-mediated rate enhancement have been reviewed in the literature [6] , [7] . Recently, an additional site-specific small self-cleaving ribozyme, termed ‘twister’, has been identified from a bioinformatics search of noncoding RNA data bases [27] . One class of twister ribozymes is composed of four helical stems labelled P1 to P4, two internal loops and one hairpin loop, as well as two predicted pseudoknots, labelled T1 and T2 ( Supplementary Results , Supplementary Fig. 1 ) [27] . Ten highly conserved nucleotides restricted to loops 1 and 4 within the twister ribozyme sequence are highlighted in red in Supplementary Fig. 1 . Cleavage chemistry required Mg 2+ cation and self-cleavage during transcription at the U5-A6 step generated products containing 2′,3′-cyclic phosphate (at U5) and 5′-OH (at A6) ends [27] . Mutations of highly conserved nucleotides (shown in red in Supplementary Fig. 1 ) or disruption of stems P1, P2 and P4, as well as the pair of pseudoknots, resulted in strong reduction in catalytic activity [27] . Further, the observed lack of cation selectivity suggested a structural rather than a catalytic role for divalent cations in twister-mediated cleavage chemistry [27] . Our efforts have focused on the twister ribozyme termed env22 ( type P1 ), whose secondary structure is shown in Fig. 1a . We have generated this twister ribozyme by annealing two chemically synthesized RNA strands, the shorter one of which is a 19-mer (residues 1–19) containing a dU5 at the U5-A6 cleavage site, whereas the longer one is a 37-mer (residues 20–56), as shown schematically in Fig. 1a . 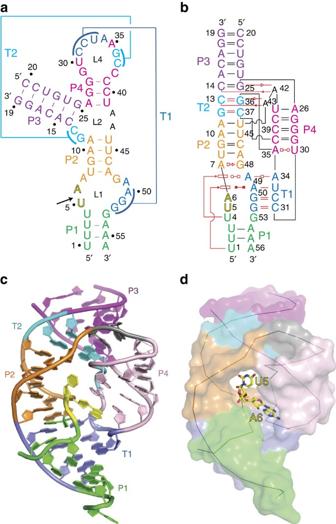Figure 1: Schematics of the secondary structure and the 2.9 crystal structure of the dU5-containingenv22 twister ribozyme. (a) A schematic of the secondary fold of theenv22twister ribozyme composed of a 19-mer substrate strand containing dU5 at the U5-A6 cleavage site. The sequence is colour-coded according to helical segments observed in the tertiary structure. Two proposed pseudoknot segments are labelled as T1 and T2. (b) A schematic of the tertiary fold observed in the crystal structure of theenv22twister ribozyme. The red lines indicate tertiary pairing. The geometric nomenclature and classification of RNA is adopted from ref.34. (c) A ribbon view of the 2.9 Å structure of theenv22twister ribozyme colour-coded as shown inaandb. (d) The same view as incbut with the RNA in a surface representation except for the U5-U6 step, which is shown in a stick representation. Figure 1: Schematics of the secondary structure and the 2.9 crystal structure of the dU5-containing env2 2 twister ribozyme. ( a ) A schematic of the secondary fold of the env22 twister ribozyme composed of a 19-mer substrate strand containing dU5 at the U5-A6 cleavage site. The sequence is colour-coded according to helical segments observed in the tertiary structure. Two proposed pseudoknot segments are labelled as T1 and T2. ( b ) A schematic of the tertiary fold observed in the crystal structure of the env22 twister ribozyme. The red lines indicate tertiary pairing. The geometric nomenclature and classification of RNA is adopted from ref. 34 . ( c ) A ribbon view of the 2.9 Å structure of the env22 twister ribozyme colour-coded as shown in a and b . ( d ) The same view as in c but with the RNA in a surface representation except for the U5-U6 step, which is shown in a stick representation. Full size image Structure of the twister ribozyme We have solved the crystal structure of the bimolecular construct of the dU5-containing env22 twister ribozyme at 2.9 Å resolution. The protocol for refinement using Phenix.refine is outlined in the Methods section. The secondary structure fold is shown schematically in Fig. 1b and the tertiary structure is shown in Fig. 1c (X-ray statistics in Table 1 and two alternate stereo views of the structure in Supplementary Fig. 2a,b ). The crystals belong to space group P6 1 22, with three molecules in the asymmetric unit, with molecule A exhibiting the best well-defined density. The three molecules adopt very similar structures; they can be superposed with pairwise root mean square deviation (RMSD) values of 0.56 Å (molecules A and B) and 1.26 Å (molecules A and C) for all atoms. Table 1 Crystallographic statistics for env22 twister ribozyme Full size table We observe formation of two pseudoknots, one of which labelled T2 involves two Watson–Crick base pairs as predicted previously [27] , whereas the other labelled T1 involves three Watson–Crick base pairs as predicted previously [27] together with an unanticipated non-canonical trans -Watson–Crick A34·A49 pair ( Fig. 1b ). We observe continuous stacking of stem P1 (in green), pseudoknot stem T1 (in blue), stem P2 (in orange), pseudoknot stem T2 (in cyan) and stem P3 (in purple; Fig. 2a ). Base pair stacking and twist between adjacent pairs at helical junctions are shown as boxed segments in Fig. 2b–e . Stem P4 (in pink) projects at an angle from the above-mentioned continuous P1-T1-P2-T2-P3 helical array ( Figs 1c and 3a ). These alignments result in a compact overall architecture with the splayed out U5-A6 step (shown in yellow) positioned in the centre of the fold ( Fig. 1d ). 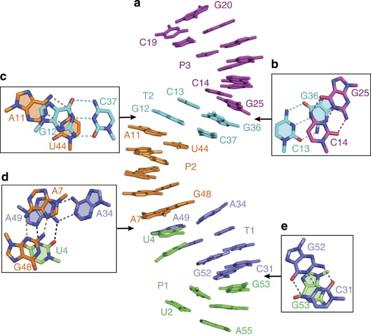Figure 2: Continuous stacking of canonical and pseudoknot stem segments in the tertiary structure of the dU5-containingenv22 twister ribozyme. (a) The continuous stacking of stem P1, pseudoknot stem T1, stem P2, pseudoknot stem T2 and stem P3 (on proceeding from bottom to top). (b–e) Stacking of adjacent base pairs at the junction of helical stems. Stacking between Watson–Crick G25-C14 (P3) and G36-C13 (T2) pairs (b), between Watson–Crick G12-C37 (T2) and A11-U44 (P2) pairs (c), between non-canonical shearedcis-Hoogsteen-sugar edge A7·G48 andtrans-Watson–Crick A34·A49 pairs (d), and between Watson–Crick G52-C31 pair and G53 (e). Figure 2: Continuous stacking of canonical and pseudoknot stem segments in the tertiary structure of the dU5-containing env2 2 twister ribozyme. ( a ) The continuous stacking of stem P1, pseudoknot stem T1, stem P2, pseudoknot stem T2 and stem P3 (on proceeding from bottom to top). ( b – e ) Stacking of adjacent base pairs at the junction of helical stems. Stacking between Watson–Crick G25-C14 (P3) and G36-C13 (T2) pairs ( b ), between Watson–Crick G12-C37 (T2) and A11-U44 (P2) pairs ( c ), between non-canonical sheared cis -Hoogsteen-sugar edge A7·G48 and trans -Watson–Crick A34·A49 pairs ( d ), and between Watson–Crick G52-C31 pair and G53 ( e ). 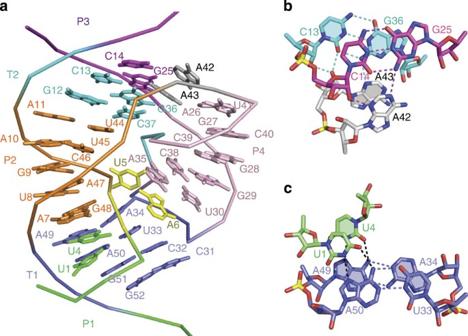Figure 3: Formation of pairs of stacked base in the structure of the dU5-containingenv22twister ribozyme. (a) Alignment of P4 relative to the T2-P2-T1 continuous helical segment. The U5-A6 step at the cleavage site is shown in yellow. (b) Stacking of A42·(C14-G25) and A43·(C13-G36) (shaded) A-minor triples. (c) Stacking of U1·(A50-U33) and U4·(A49-A34) (shaded) major groove triples. Full size image Figure 3: Formation of pairs of stacked base in the structure of the dU5-containing env22 twister ribozyme. ( a ) Alignment of P4 relative to the T2-P2-T1 continuous helical segment. The U5-A6 step at the cleavage site is shown in yellow. ( b ) Stacking of A42·(C14-G25) and A43·(C13-G36) (shaded) A-minor triples. ( c ) Stacking of U1·(A50-U33) and U4·(A49-A34) (shaded) major groove triples. Full size image Base triple-mediated tertiary interactions A set of tertiary interactions involving two pairs of stacked base triples ( Fig. 3b,c ; Supplementary Fig. 3a–d ) and three non-canonical base pairs ( Supplementary Fig. 3d–f ) contribute to the overall fold of the twister ribozyme. Thus, A42 and A43 within the upper internal loop ( Fig. 1a ) participate in stacked A42·(C14-G25) ( Supplementary Fig. 3a ) and A43·(C13-G36) ( Supplementary Fig. 3b ) minor groove base triples ( Fig. 3b ) that stabilize the junctional pairs connecting stem P3 and pseudoknot stem T2 ( Fig. 1b,c ). In addition, nucleotides U1 and U4 at either end of stem P1 ( Fig. 1a ) form stacked U1·(U33-A50) ( Supplementary Fig. 3c ) and U4·(A34·A49) ( Supplementary Fig. 3d ) major groove base triples ( Fig. 3c ) that stabilize junctional pairs involved in continuous stacking of pseudoknot stem T1 with stem P2 ( Fig. 1b,c ). Notably, both A34 and A49 involved in non-canonical trans -Watson–Crick pairing ( Supplementary Fig. 3d ) are highly conserved in twister ribozymes ( Supplementary Fig. 1 ). Finally, stem P2 is extended by formation of a sheared cis -Hoogsteen-sugar edge A7·G48 pair ( Supplementary Fig. 3e ), whereas the hairpin loop zippers up further by formation of Watson–Crick G29-C38 and non-canonical trans- Watson–Crick-Hoogsteen U30·A35 ( Supplementary Fig. 3f ) pair. Notably, A7, G29, U30, A35, C38 and G48 involved in the above pairing alignments are highly conserved nucleotides in twister ribozymes ( Supplementary Fig. 1a ). Thus, all internal and hairpin loop bases are involved in pairing interactions (non-canonical pairs, base triples and pseudoknot-based pairing) except for the bases U5 and A6 centred at the cleavage site. Splayed-out U5-A6 conformation at cleavage step We observe segments within the overall fold in our structure of the twister ribozyme where adjacent bases adopt a splayed-out conformation. One such segment spans U4-U5-A6-A7, where splayed conformations are observed at U4-U5, U5-A6 cleavage site and A6-A7 steps ( Supplementary Fig. 4a ). Another such segment spans A34-A35-G36-C37-C38, where all adjacent bases adopt a splayed conformation, except for the stacked G36-C37 step ( Supplementary Fig. 4b ). Note that also non-adjacent A35 and C38 are also stacked on each other. The twister ribozyme fold centered about the U5-A6 step (in yellow) is shown in stereo in Fig. 4a . The U5-A6 step associated with the cleavage site adopts an extended splayed out conformation with the base edges at either end anchored by hydrogen bonding to backbone phosphates. Thus, the N3H of U5 is hydrogen bonded to the non-bridging oxygen of the U44-U45 phosphate, whereas the NH 2 -6 of A6 is hydrogen bonded to the non-bridging oxygen of the C31-C32 phosphate ( Fig. 4b ). In addition, the base of A6 adopts a syn alignment stabilized through stacking with the highly conserved non-canonical trans -Watson–Crick-Hoogsteen U30·A35 pair, whereas its 2′-OH is hydrogen bonded to N3 of highly conserved A34 ( Fig. 4b ). Thus, the base and sugar of highly conserved A6 are anchored in place by stacking and hydrogen bonding interactions. By contrast, U5, which is not conserved among twister ribozymes, exhibits no stacking interactions and a single intermolecular contact mentioned above. The sugar pucker geometries are C3′- endo for U5 and C2′- endo for A6. 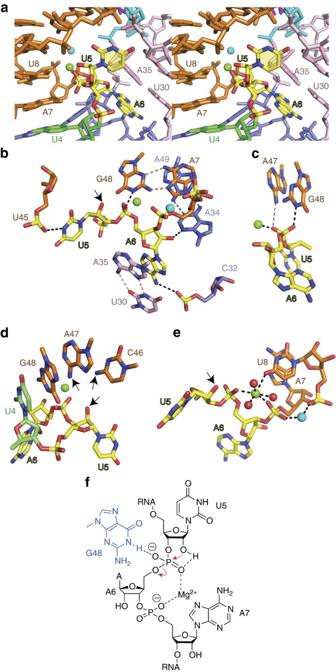Figure 4: Intermolecular contacts and bound metal ions at the U5-A6 cleavage site step in the structure of the dU5-containingenv22twister ribozyme and chemical drawing showing the structure-derived, chemically important entities for theenv22ribozyme self-cleavage mechanism. (a) A stereo view of the U5-A6 step (in yellow) nestled within the major groove of stem P2 (in orange). Bound Mg2+and an unassigned cation within the U5-A6-A7 segment are shown in green and cyan. (b) A view of intermolecular hydrogen bonds involving the U5-A6 step. Also shown is the relative positioning of A7·G48, U30·A35 and A34·A49 non-canonical pairs. (c) View showing hydrogen bonding by A47 (weak) and G48 (strong) and coordination by bound Mg2+cation to the non-bridging oxygens of the phosphate at the U5-A6 step. (d) View showing the positioning of G48 directed towards the non-bridging oxygens of the phosphate at the U5-A6 step, and the positioning of C46 and A47 directed towards the modelled 2′-O of U5. Arrows indicate amino groups of C46 and A47 that are directed towards the 2′-O of U5. (e) Bound cations at the U5-A6-A7 step. The bound Mg2+and unassigned cation are in green and cyan, respectively, whereas water molecules are in red. (f) Schematic highlighting in-line attack of the U5 2′-OH, Mg2+coordination to U5-A6 and A6-A7 phosphodiester groups. Figure 4: Intermolecular contacts and bound metal ions at the U5-A6 cleavage site step in the structure of the dU5-containing env22 twister ribozyme and chemical drawing showing the structure-derived, chemically important entities for the env22 ribozyme self-cleavage mechanism. ( a ) A stereo view of the U5-A6 step (in yellow) nestled within the major groove of stem P2 (in orange). Bound Mg 2+ and an unassigned cation within the U5-A6-A7 segment are shown in green and cyan. ( b ) A view of intermolecular hydrogen bonds involving the U5-A6 step. Also shown is the relative positioning of A7·G48, U30·A35 and A34·A49 non-canonical pairs. ( c ) View showing hydrogen bonding by A47 (weak) and G48 (strong) and coordination by bound Mg 2+ cation to the non-bridging oxygens of the phosphate at the U5-A6 step. ( d ) View showing the positioning of G48 directed towards the non-bridging oxygens of the phosphate at the U5-A6 step, and the positioning of C46 and A47 directed towards the modelled 2′-O of U5. Arrows indicate amino groups of C46 and A47 that are directed towards the 2′-O of U5. ( e ) Bound cations at the U5-A6-A7 step. The bound Mg 2+ and unassigned cation are in green and cyan, respectively, whereas water molecules are in red. ( f ) Schematic highlighting in-line attack of the U5 2′-OH, Mg 2+ coordination to U5-A6 and A6-A7 phosphodiester groups. Full size image The N1H of G48 forms a hydrogen bond (heteroatom separation of 2.6 Å) to the non-bridging pro-R phosphate oxygen, whereas NH 2 of A47 forms a weaker hydrogen bond (heteroatom separation of 3.5 Å) to the non-bridging pro-S phosphate oxygen at the U5-A6 cleavage site ( Fig. 4c ). Three alternate views of the omit electron density maps (3 σ ) for the U5-A6 step and bases C46, A47 and G48 are shown in Supplementary Fig. 5 . We also compare omit electron density maps (3 σ ) for a single view of the catalytic pocket of the three molecules in the asymmetric unit in Supplementary Fig. 6 . Bound metal ions A bound cation (green ball, Fig. 4 ) is directly coordinated to non-bridging pro-S and pro-R phosphate oxygens of the U5-A6 (distance 2.2 Å) and A6-A7 (distance 2.2 Å) steps, respectively, to the O4 carbonyl oxygen of U8, and three water molecules (red balls, Fig. 4e ). The bound cation was assigned to Mg 2+ following detection of density at this site in an anomalous data set collected on crystals of the ribozyme soaked in Mn 2+ solution (red arrow in Supplementary Fig. 7a–c ). Another cation (cyan ball, Fig. 4 ) is directly coordinated to the non-bridging pro-S and pro-R phosphate oxygens of the A6-A7 and A7-U8 steps, respectively. We are uncertain on whether this is a monovalent or divalent cation as no anomalous signal was observed at this site in Mn 2+ -soaked crystals of the twister ribozyme. The separation between these two bound cations is 6.2 Å. Additional divalent Mg 2+ cations bridge the backbone phosphates of RNA segments aligned in close proximity (black arrows in Supplementary Fig. 7a,b,d,e ). Modelling of the putative nucleophilic 2′-OH of U5 Our structure of the twister ribozyme contained a 2′-H at U5 (dU5), so as to prevent self-cleavage at the U5-A6 step by an active ribozyme. Following structure refinement, the 2′-H was modelled by 2′-OH at U5, to check for in-line alignment required for cleavage of the P-O5′ bond of the intervening phosphate at the U5-A6 step. The modelled 2′-OH structure exhibited a 2′-O (of U5) to P (at U5-A6 step) distance of approximately 2.8 Å and a 2′-O (of U5) to P-O5′ angle (at U5-A6 step) of approximately 148°( Fig. 4d ). There were no heteroatoms within 4.0 Å of the modelled 2′-O of U5 in the structure of the complex. However, the NH 2 nitrogen of A47 and the NH 2 nitrogen of C46 are directed towards the 2′-O of U5 with heteroatom separations of 4.2 and 4.1 Å, respectively ( Fig. 4d ). Mutations and cleavage activities We performed cleavage assays of several single-nucleotide twister variants using ion-exchange high-performance liquid chromatography (HPLC; Fig. 5 and Supplementary Fig. 8 ). As expected, mutations of the non-conserved U5, to A5 or G5, showed activities comparable to the WT sequence. However, nucleosides that were involved in significant recognition patterns such as A6 (NH 2 -6 hydrogen bonded to C31-C32 phosphate) or G48 (N1H-hydrogen bonded to scissile phosphate) were highly sensitive to mutations, with A6G completely abolishing cleavage, and G48A reducing cleavage to a very minor fraction ( Fig. 5 ). Of note, mutations of A47 (NH 2 -6 directed towards the 2′-O of U5) to G47, or C46 (NH 2 -4 directed towards the 2′-O of U5) to U46, exhibited reduced ribozyme activities ( Supplementary Fig. 8 ). The U8C mutation with the heteroatom-4 pyrimidine position close to the Mg 2+ site showed only minimal reduction in cleavage propensity ( Supplementary Fig. 8 ). 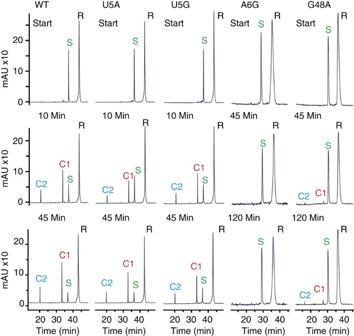Figure 5: Self-cleavage of theenv22twister ribozyme mutants U5A, U5G, A6G and G48A. Cleavage analysed at 40 μM RNA each strand; 2 mM MgCl2, 100 mM KCl, 30 mM HEPES, pH 7.5, 23 °C. R 37-nt ribozyme, S 19-nt substrate; C1 and C2, 14-nt and 5-nt cleavage products. HPLC conditions: Dionex DNAPac column (4 × 250 mm2), 80 °C, 1 ml min−1, 0–60% buffer B in 45 min. Buffer A: Tris–HCl (25 mM), urea (6 M), pH 8.0. Buffer B: Tris–HCl (25 mM), urea (6 M), NaClO4(0.5 M), pH 8.0. Figure 5: Self-cleavage of the env22 twister ribozyme mutants U5A, U5G, A6G and G48A. Cleavage analysed at 40 μM RNA each strand; 2 mM MgCl 2 , 100 mM KCl, 30 mM HEPES, pH 7.5, 23 °C. R 37-nt ribozyme, S 19-nt substrate; C1 and C2, 14-nt and 5-nt cleavage products. HPLC conditions: Dionex DNAPac column (4 × 250 mm 2 ), 80 °C, 1 ml min −1 , 0–60% buffer B in 45 min. Buffer A: Tris–HCl (25 mM), urea (6 M), pH 8.0. Buffer B: Tris–HCl (25 mM), urea (6 M), NaClO 4 (0.5 M), pH 8.0. Full size image Fluorescence assays: kinetics and conformational changes We utilized a fluorescence-based, real-time cleavage assay [28] , [29] to monitor cleavage kinetics ( Fig. 6 ). Therefore, 2-aminopurine (AP) was integrated into one of the two base pairs of stem P1 (U3AP–A54U). AP is expected to become stacked (and hence fluorescence-quenched) upon formation of the P1 stem on addition of Mg 2+ . Upon cleavage, however, the 5-nt cleavage product should dissociate fast because of the very weak base pairing interactions. Indeed, cleavage resulted in a significant fluorescence increase that was attributed to the release of the AP containing pentamer. The fluorescence trace was fitted to a single-exponential equation yielding k obs =2.44±0.31 min −1 at pH 7.5 and 20 °C. This value decreased to 1.41±0.16 min −1 when the temperature was lowered to 15 °C ( Fig. 6c,d ). Lowering the temperature further to 10 °C ( Fig. 6e ) manifested in biexponential behaviour indicating that, likely, slow dissociation of the cleavage product has to be taken into account as a rate-limiting step. We furthermore showed that the apparent cleavage rate was reduced about 1.5-fold when the pH value was lowered to 7.0 or 6.5 ( Fig. 6f ). 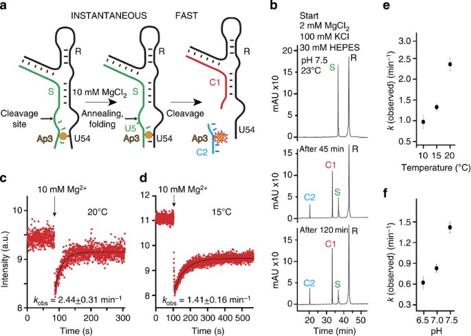Figure 6: Cleavage kinetics of theenv22twister ribozyme analysed by 2-aminopurine fluorescence. (a) Schematics of the assay indicating AP position, P1 folding and cleavage product release. (b) Cleavage of the U3AP–A54U variant analysed by HPLC (for conditions see caption ofFig. 5). (c) Fluorescence response of the U3AP–A54U variant upon MgCl2addition; conditions:cRNA=0.3 mM, 50 mM potassium 3-(N-morpholino)propanesulfonate (KMOPS), 100 mM KCl, 20 °C, pH 7.5; mixing was performed manually in less than 2 s resulting in 10 mM Mg2+concentration. (d) Same asc, but 15 °C. (e) Plot of apparent rateskobsversus temperature. (f) Plot of apparent rateskobsversus pH value. Figure 6: Cleavage kinetics of the env22 twister ribozyme analysed by 2-aminopurine fluorescence. ( a ) Schematics of the assay indicating AP position, P1 folding and cleavage product release. ( b ) Cleavage of the U3AP–A54U variant analysed by HPLC (for conditions see caption of Fig. 5 ). ( c ) Fluorescence response of the U3AP–A54U variant upon MgCl 2 addition; conditions: c RNA =0.3 mM, 50 mM potassium 3-( N -morpholino)propanesulfonate (KMOPS), 100 mM KCl, 20 °C, pH 7.5; mixing was performed manually in less than 2 s resulting in 10 mM Mg 2+ concentration. ( d ) Same as c , but 15 °C. ( e ) Plot of apparent rates k obs versus temperature. ( f ) Plot of apparent rates k obs versus pH value. Full size image Importantly, cleavage in our assays was initiated by the addition of Mg 2+ at saturating concentrations of 10 mM. This concentration guarantees that folding of the ribozyme into the catalytically active conformation occurs almost instantaneously (in less than 1–2 s corresponding to the immediate fluorescence decrease that is consistent with AP3·U54 base pair stabilization; Fig. 6c,d ). Independent evidence for this rapid folding process stems from an A5AP twister ribozyme variant that showed immediate fluorescence increase upon Mg 2+ addition, suggesting the conformational rearrangement into an unstacked position of the nucleoside in position 5 ( Supplementary Fig. 9 ) as observed in the crystal structure. The A5AP variant surprisingly shows significantly slower cleavage (see HPLC cleavage assay in Supplementary Fig. 9b ), and hence allowed an analysis of the adaption of nucleoside-5 into a cleavage-relevant conformation with respect to varying Mg 2+ concentrations. To achieve this conformation, concentrations higher than 1 mM Mg 2+ were required. Interestingly, monovalent K + cation alone could not cause a comparable effect ( Supplementary Fig. 9c,d ). In addition, we investigated an A6AP variant ( Supplementary Fig. 10 ). As expected, this mutation does not show cleavage (which is consistent with the deleterious A6G mutation, Fig. 5 ), hence highlighting again the importance of hydrogen bond formation between the NH 2 -6 proton and the C31-C32 (2.8 Å) phosphate. It should be noted that the little but significant fluorescence increase upon addition of millimolar Mg 2+ concentrations indicates that nucleoside-6 becomes more solvent-accessible (and less fluorescence-quenched) in response to the outward-directed conformational flip of the neighbouring nucleoside-5 on Mg 2+ addition (compare schematics in Fig. 6a and Supplementary Fig. 10 ). Small nucleolytic ribozymes are widespread within noncoding RNAs across genomes at the cellular level. Our structure of the widely distributed (from bacteria to plants and metazoans) twister ribozyme adds a distinct architecture to the limited database of structures of small non-cleaving ribozymes that include the hammerhead [12] , [13] , [14] , hairpin [15] , [16] , [17] , [18] , glmS [19] , [20] , [21] , hepatitis delta virus [10] , [22] , [23] , [24] and Varkud Satellite [25] ribozymes involved in gene regulation. The twister ribozyme adopts a novel tertiary fold generated through co-linear stacking of helical stems, formation of a pair of pseudoknots, two minor groove and two major groove base triples and two-long range non-canonical pairs ( Fig. 1b,c ). Strikingly, interdigitation of the canonical (P1, P2 and P3) and pseudoknot (T1 and T2) helical stems results in formation of a continuous helical architecture ( Fig. 2 ). Formation of pseudoknots T1 and T2 position a segment of the hairpin loop and stem P4 in the vicinity of the U5-A6 cleavage site ( Fig. 1c ). There are ten highly conserved nucleotides in the twister ribozyme identified from phylogenetic studies ( Supplementary Fig. 1a ). Of these, six (A7, U30, A34, A35, G48 and A49) are involved in the formation of sheared cis -Hoogsteen-sugar edge A7·G48, trans- Watson–Crick-Hoogsteen U30·A35 and trans -Watson–Crick A34·A49 non-canonical pairs, which are located in the vicinity of the U5-A6 cleavage site in the tertiary structure of the ribozyme ( Fig. 4b ). Of the remaining four (A6, G29, G36, C38) conserved nucleotides ( Supplementary Fig. 1 ), A6 is part of the cleavage site, G29 and C38 form a Watson–Crick pair, as do G36 and C13, with the G29-C38 pair, also positioned in the vicinity of the cleavage site ( Fig. 3a ). We observe a splayed alignment at the U5-A6 step, with A6 in a syn conformation, and the sugar puckers adopting a U5(C3′- endo )-A6(C2′- endo ) pucker orientation. A6 is held in a more rigid orientation than U5, given that its base stacks with the U30·A35 non-canonical pair and its sugar 2′-OH is hydrogen-bonded to the minor groove edge of A34 ( Fig. 4b ). Importantly, its NH 2 -6 group forms a direct hydrogen bond with the C31-C32 phosphate, with disruption of this hydrogen bond following mutations to G6 or AP6 abolishing activity ( Fig. 4b ). We note that the modelled 2′-O of U5 is positioned for in-line cleavage of the P-O5′ bond without any conformational changes required to achieve this catalytically competent state. Unexpectedly, we identified a Mg 2+ cation coordinated to the non-bridging phosphate oxygens of the U5-A6 and A6-A7 steps, whereas an unassigned cation was coordinated to the non-bridging phosphate oxygens of the A6-A7 and A7-U8 steps ( Fig. 4e ). These cations most likely contribute to the structural integrity of the twister ribozyme at and in the vicinity of the cleavage site. Several bases are directed towards the 2′-O of U5 (C46 and A47; Fig. 4d ), towards the non-bridging phosphate oxygen at the U5-A6 step (A47 and G48; Fig. 4c ) and towards the Mg 2+ cation (U8; Fig. 4e ). Interestingly, for these nucleosides, mutations were largely tolerated in position 8, resulted in reduced cleavage activity at positions 46 and 47, whereas only mutation in position 48 was fully deleterious ( Fig. 5 and Supplementary Fig. 6 ), emphasizing the key role of G48 in the catalytic mechanism. We do not have a ready explanation as to why the U8C mutation had no major impact on cleavage activity. There are currently two main mechanisms of RNA-mediated catalysis, with the majority of self-cleaving ribozymes adopting the general nucleolytic acid–base catalysis pathway, whereas self-splicing introns and RNase P act as metalloenzymes [30] . There are no bases within direct hydrogen bond distance of the 2′-O of U5, but the NH 2 of A47 (purines are conserved at this position [27] ) and NH 2 of C46 (pairing is highly conserved at the 9–46 base pair position [27] ) are within water-mediated hydrogen-bonding distance ( Fig. 4c ). Their potential contribution to catalysis requires further investigation given that C46U and A47G mutants result in reduced but not abolished catalytic activity ( Supplementary Fig. 8 ). The N1H of highly conserved G48 forms a direct hydrogen bond to the non-bridging pro-R phosphate oxygen of the U5-A6 step ( Fig. 4c ) and hence is a strong candidate for stabilization of the transition state in the reaction pathway. Strongly reduced cleavage observed for the G48A mutant supports such a scenario ( Fig. 5 ). Earlier biochemical studies on the twister ribozyme ruled out direct participation of divalent metal ions in the cleavage mechanism, and assigned the requirement for Mg 2+ to a structural rather than a catalytic role [27] . However, we observe a Mg 2+ bound to the non-bridging pro-S phosphate oxygen at the U5-A6 cleavage site in our structure of the twister ribozyme, placing it in a position where it has the potential to provide electrostatic stabilization of the developing negative charge on the scissile phosphate following the cleavage of the P-O5′ bond. Nevertheless, given that the biochemical data are not in favour of a direct participation of the Mg 2+ in the cleavage mechanism [27] , it appears that its primary contribution must be to the structural integrity of the cleavage site. Our real-time fluorescence-based cleavage assay revealed cleavage kinetics for the twister ribozyme ( Fig. 6 ) that are consistent with the previously reported observed rates in the range of 1–10 min −1 , as well as the same trend for pH dependencies [27] , [31] . Importantly, we show that temperature has a significant impact on the observed rates ( Fig. 6e ), which likely correlates to multiple factors, including proper folding of the P1 stem, conformational rearrangement of the nucleoside-5 into an unstacked and splayed out position in response to Mg 2+ ( Supplementary Fig. 9 ), but also to release of the cleavage product. The slightly reduced cleavage rate when lowering the pH may reflect a destabilization of the hydrogen bond formed between G48-N1H and one of the non-bridging oxygens of the scissile phosphate [31] . It has been pointed out to us that the twister ribozyme shares similarities with the hairpin ribozyme, with both hairpin and twister ribozymes having a syn purine and a C2′-endo sugar at the +1 position. The catalytic pockets of the hairpin and env22 twister ribozymes are compared in Supplementary Fig. 11 . Recently, there has been a report of a 2.3 Å crystal structure of the twister ribozyme from Oryza sativa [32] . The construct in this study is distinct from the env22 twister ribozyme in that it lacks stem P3, and in addition contains a fully paired stem P1. At the global level, the O. sativa [32] and env22 (this study) twister ribozymes adopt similar folds stabilized by the same dual-pseudoknot and non-canonical pairing interactions, as well as the alignment of the anchored A base (intermolecular hydrogen bonds, stacking, syn alignment and sugar pucker) at the U-A cleavage site. One important difference between the two ribozymes is in stem P1, wherein pairing within the (U1-U2-U3-U4) and (G53-A54-A55-A56) of the env22 twister ribozyme is restricted to U2-A55 and U3-A54 Watson–Crick pairs, whereas U1 and U4 do not pair with A56 and G53, respectively, but instead participate in the formation of two base triples ( Fig. 1b and Supplementary Fig. 3c,d ). By contrast, stem P1 in the O. sativa ribozyme [32] forms five Watson–Crick G-C pairs, precluding base pair disruption and the formation of the two base triples around the active site. Interestingly, very similar base triples could be formed involving cytosines at positions C1 and C4. A major and critical difference between the structures of the two ribozymes is related to alignment of the U base/sugar at the U-A cleavage site. Thus, although the modelled O2′ oxygen of U5 is positioned for near in-line targeting of the to-be-cleaved P-O bond (O2′ of U to P-O5′ distance of 2.8 Å and angle of 148°) at the U5-A6 step in the env22 twister ribozyme ( Fig. 7a , this study), the corresponding modelled O2′ oxygen adopts an off-line orthogonal alignment (O2′ of U to P-O5′ distance of 4.1 Å and angle of approximately 83°) from that required for in-line cleavage in the O. sativa ribozyme (PDB: 40JI; Fig. 7b ) [32] . Further, although a Mg 2+ is directly coordinated to the non-bridging cleavable phosphate oxygen in the env22 twister ribozyme (this study), no corresponding divalent cation was observed at the cleavage site in the structure of the O. sativa ribozyme [32] . 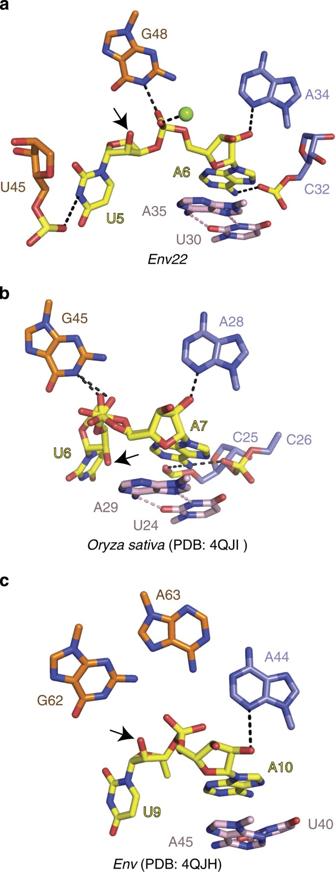Figure 7: Comparison ofenv22(this study),O. sativa(4OJI) andenv(4QJH) twister ribozymes. (a) In-line alignment of the U-A step in the 2.9 Å structure of theenv22twister ribozyme with the emphasis on the position of the modelled 2′-O of U relative to the adjacent P-O5′ bond. (b) Off-line orthogonal alignment of the U-A step in the 2.3 Å structure of theO. sativatwister ribozyme (PDB: 4OJI). (c) Off-line orthogonal alignment of the U-A step in the 4.1 Å structure of theenvtwister ribozyme (PDB: 4QJH). Figure 7: Comparison of env22 (this study), O. sativa (4OJI) and env (4QJH) twister ribozymes. ( a ) In-line alignment of the U-A step in the 2.9 Å structure of the env22 twister ribozyme with the emphasis on the position of the modelled 2′-O of U relative to the adjacent P-O5′ bond. ( b ) Off-line orthogonal alignment of the U-A step in the 2.3 Å structure of the O. sativa twister ribozyme (PDB: 4OJI). ( c ) Off-line orthogonal alignment of the U-A step in the 4.1 Å structure of the env twister ribozyme (PDB: 4QJH). Full size image The absence of an in-line alignment in the structure of the O. sativa ribozyme could be resolved through incorporation of a sizeable conformational change in the U base at the U-A cleavage site so as to position its O2′ for in-line attack [32] . The rationale for the proposed conformational change was that the U base at the U-A cleavage site was involved in packing interactions and needed to be repositioned to facilitate in-line alignment. It remains to be established to what extent formation of a five-base pair P1 stem, by preventing the formation of two base triples, perturbed completion of the active site and the geometry of the U base at the U-A cleavage step, as well as contributing to the absence of a Mg 2+ cation at the cleavage site in the structure of the O. sativa ribozyme 32 . Both structures of the O. sativa [32] and env22 (this study) twister ribozymes highlight the important contribution of the same guanine (G48 in the env22 twister ribozyme, this study) to acid–base catalysis, with the additional emphasis in this study for Mg 2+ at the cleavage site in the env22 twister ribozyme playing a structural role. A second group has also recently reported on two structures of the twister ribozyme [33] . One of these structures is for the O. sativa twister ribozyme at 3.1 Å resolution (4QJD), which could not provide insights into the catalytic mechanism given that it exhibits a disordered scissile phosphate and nucleotide 5′ to the cleavage site [33] . The other structure is for an environmental ( env ) twister ribozyme at 4.1 Å resolution (4QJH) where the O2′ linkage is positioned in an off-line orthogonal alignment in relation to the scissile phosphate (O2′ of U to P-O5′ distance of 2.9 Å and angle of 83° for molecule A of three molecules in the asymmetric unit; the other two molecules show angles of 107° and 87°) [33] . The alignment of residues at the active site relative to the scissile phosphate is shown in Fig. 7c . These include a guanosine proposed to deprotonate the 2′-OH of the nucleotide 5′ to the cleavage site (heteroatom-heteroatom separation of 4.7 Å) and an adenosine that could neutralize the negative charge on the non-bridging phosphate oxygen (heteroatom-heteroatom separation of 3.7 Å) at the cleavage site. Stem P1 for this env twister ribozyme contained eight base pairs precluding formation of the base triples identified in our study of the env22 twister ribozyme. The paper did not report on the presence of a divalent cation at the cleavage site, nor could one have been definitively identified at 4.1 Å resolution. In conclusion, the off-line orthogonal alignments in the 2.3 Å structure of the O. sativa twister ribozyme (O2′ to P-O5′ angle: 83 ° ; 4OJI) [32] and the 4.1 Å structure of the env twister ribozyme (angle: 83 ° ; 4QJH) [33] , contrasts with the near in-line alignment (angle: 148 ° ) observed in the 2.9 Å structure of the env22 twister ribozyme reported in this study ( Fig. 7 ). A disquieting feature of these structures reflects the different positioning of key residues lining the cleavage site ( Fig. 7a–c ), and the absence/presence of a divalent cation at the cleavage site ( Fig. 7a–c ). On the other hand all three structures emphasized a key role for the same invariant guanosine in catalysis. Further experimentation on in-line complexes at higher resolution is required to resolve these contrasting views of alignments within the cleavage site between the three crystal structures of the twister ribozyme. Solid-phase synthesis of oligoribonucleotides Standard phosphoramidite chemistry was applied for RNA solid-phase synthesis using 2′- O -TOM nucleoside phosphoramidite building blocks (ChemGenes) and polystyrene support (GE Healthcare, Custom Primer SupportTM, 80 μmol g −1 ; PS 200). All oligonucleotides were synthesized on a ABI 392 Nucleic Acid Synthesizer following standard methods: detritylation (80 s) with dichloroacetic acid/1,2-dichloroethane (4/96); coupling (2.0 min) with phosphoramidites/acetonitrile (0.1 M × 130 μl) and benzylthiotetrazole/acetonitrile (0.3 M × 360 μl); capping (3 × 0.4 min, Cap A/Cap B=1/1) with Cap A: 4-(dimethylamino)pyridine in acetonitrile (0.5 M) and Cap B: Ac 2 O/sym-collidine/acetonitrile (2/3/5); oxidation (1.0 min) with I 2 (20 mM) in tetrahydrofuran (THF)/pyridine/H 2 O (35/10/5). The solutions of amidites and tetrazole, and acetonitrile were dried over activated molecular sieves (4 Å) overnight [35] . 5′- O -(4,4′-Dimethoxytrityl)-2′-deoxyuridine phosphoramidite was purchased from ChemGenes. 5′- O -(4,4′-dimethoxytrityl)-2′- O -[(triisopropylsilyl)oxy]methyl-2-AP phosphoramidite was synthesized according to ref. 35 . Deprotection of oligonucleotides The solid support was treated each with MeNH 2 in EtOH (33%, 0.5 ml) and MeNH 2 in water (40%, 0.5 ml) for 7 h at room temperature. The supernatant was removed from and the solid support was washed 3 × with ethanol/water (1/1, v/v). The supernatant and the washings were combined and the whole mixture was evaporated to dryness. To remove the 2′-silyl-protecting groups, the resulting residue was treated with tetrabutylammonium fluoride trihydrate (TBAF·3H 2 O) in THF (1 M, 1 ml) at 37 °C overnight. The reaction was quenched by the addition of triethylammonium acetate (1 M, pH 7.4, 1 ml). The volume of the solution was reduced and the solution was desalted with a size exclusion column (GE Healthcare, HiPrep 26/10 Desalting; 2.6 × 10 cm; Sephadex G25) eluting with H 2 O, the collected fraction was evaporated to dryness and dissolved in 1 ml H 2 O. Analysis of the crude RNA after deprotection was performed by anion-exchange chromatography on a Dionex DNAPac PA-100 column (4 × 250 mm) at 80 °C. Flow rate: 1 ml min −1 , eluant A: 25 mM Tris·HCl (pH 8.0), 6 M urea; eluant B: 25 mM Tris·HCl (pH 8.0), 0.5 M NaClO 4 , 6 M urea; gradient: 0–60% B in A within 45 min or 0–40% B in 30 min for short sequences up to 15 nucleotides, ultraviolet detection at 260 nm. Purification of RNA Crude RNA products were purified on a semipreparative Dionex DNAPac PA-100 column (9 × 250 mm) at 80 °C with flow rate 2 ml min −1 . Fractions containing RNA were loaded on a C18 SepPak Plus cartridge (Waters/Millipore), washed with 0.1–0.15 M (Et 3 NH) + HCO 3 – , H 2 O and eluted with H 2 O/CH 3 CN (1/1). RNA containing fractions were lyophilized. Analysis of the quality of purified RNA was performed by anion-exchange chromatography with same conditions as for crude RNA; the molecular weight was confirmed by liquid chromatography-electrospray ionization (LC-ESI) mass spectrometry. Yield determination was performed by ultraviolet photometrical analysis of oligonucleotide solutions. Mass spectrometry RNA All experiments were performed on a Finnigan LCQ Advantage MAX ion trap instrumentation connected to an Amersham Ettan micro LC system. RNA sequences were analysed in the negative-ion mode with a potential of −4 kV applied to the spray needle. LC: Sample (200 pmol RNA dissolved in 30 μl of 20 mM EDTA solution; average injection volume: 30 μl); column (Waters XTerraMS, C18 2.5 μm; 1.0 × 50 mm) at 21 °C; flow rate: 30 μl min −1 ; eluant A: 8.6 mM TEA, 100 mM 1,1,1,3,3,3-hexafluoroisopropanol in H 2 O (pH 8.0); eluant B: methanol; gradient: 0–100% B in A within 30 min; ultraviolet-detection at 254 nm. Crystallization The sample for crystallization was generated by annealing the purified env22 twister ribozyme at 70 °C for 3 min in a buffer containing 50 mM K-potassium 4-(2-hydroxyethyl)-1-piperazineethanesulfonic acid (HEPES), pH 6.8, 100 mM KCl and 2 mM MgCl 2 followed by incubation at room temperature for 5 min and then cooling on ice for 30 min before setting up crystallization trials. The crystals of the env22 twister ribozyme were grown at 20 °C over a period of 1 week using the sitting-drop vapour diffusion approach after mixing the RNA at an equimolar ratio with the reservoir solution containing 0.1 M imidazole, pH 7.9, CaCl 2 0.2 M and 14–16% PEG1000. For data collection, crystals were quickly transferred into a cryoprotectant solution containing 0.1 M imidazole, pH 7.9, CaCl 2 0.2 M, 20% PEG1000 and 10% glycerol and flash-frozen in liquid nitrogen. For Ir(NH 3 ) 6 3+ and Mn 2+ soaking experiments, crystals were transferred into the crystallization solution containing 0.1 M imidazole, pH 7.9, CaCl 2 0.2 M, 20% PEG1000 and supplemented with 5 mM Ir(NH 3 ) 6 3+ Cl 3 or 50 mM MnCl 2 at 4 °C for 24 h. X-ray data collection and refinement All X-ray diffraction data were collected at 100 K at NE-CAT beamline 24-ID-C located at the Advanced Photon Source, using Pilatus 6 M detector. Data were processed using the HKL2000 (HKL Research) and XDS programmes. The crystals belong to space group P6 1 22 ( Table 1 ). Based on the molecular weight of 16,000 Da, three molecules are expected per asymmetric unit with 65% solvent, which is typical for RNA molecules. Using the Iridium SAD data, six Iridium sites were located using SHELXC and SHELXD as implemented in HKL2MAP programme [36] . These heavy atom sites were refined and six additional minor sites were located using the programme PHASER. The resulting phases were then subjected to density modification using RESOLVE and PARROT. It was not possible to determine the non-crystallographic symmetry (NCS) relations using the heavy atom sites. However, most parts of a single molecule could be built. This approximate model was used to perform a phased molecular replacement using the programme MOLREP to locate three molecules and to identify the NCS relationships between them. Iterations of model building, phase combination and NCS-based density modification enabled us to build the complete model using COOT [37] . The model was refined using the 2.9 Å native data set ( Table 1 ). We modelled deoxyriboU at the cleavage site as DU, using the CCP4 monomer library for DU and default weighting in the refinement by two refinement programmes—Refmac [38] and Phenix.refine [39] . We used 20 rounds of restrained and Translation-Libration-Screw-rotation (TLS) refinement in Refmac, and three macrocycles of restrained and TLS refinement including one round of simulated annealing in refinement using Phenix.refine. Before refinement, we added link information for atoms coordinated to Mg ion so that metal–ion coordination distances could be refined based on the ideal bond/angle present in the library. Both the refinement programmes produced similar structures with comparable R and R-free, with Phenix.refine [39] producing slightly better statistics than Refmac [38] . The X-ray statistics for the structure of the env22 twister ribozyme using Phenix.refine are listed in the Table 1 . Out of three molecules in the asymmetric unit, molecule A exhibits the best well-defined electron density, with the quality decreasing on proceeding to molecule B and then to molecule C. The three molecules adopt very similar structures; they can be superposed with pairwise RMSD values of less than 1.26 Å for all atoms. The O2′ of U5 to P-O5′ of A6 angle reflecting the extent of in-line alignment was 148°, 137° and 127° for molecules A, B and C, respectively. All presentation and discussions of the structure of the env22 twister ribozyme in this paper are based on the structure of molecule A. Metal ions and their coordinated waters were identified based on 2Fo-Fc and Fo-Fc maps guided by the coordination geometries. Mg 2+ sites were identified by soaking crystals of the complex in Mn 2+ -containing solution and collecting an optimized anomalous data set. The X-ray data statistics of the native, iridium hexamine-containing and Mn 2+ -soaked crystals are listed in Table 1 . The Mn 2+ -soaked structures were refined using native twister ribozyme structure as a starting model. Cleavage assays Aliquots from aqueous millimolar stock solutions of the two RNA strands (R: ribozyme; S: substrate) were mixed and lyophilized. After addition of reaction buffer (30 mM HEPES, pH 7.5, 100 mM KCl, 2 mM MgCl 2 ) to yield a final concentration of c RNA =55 μM (each strand) in a total volume of 20 μl, the reaction was stopped by the addition of EDTA solution (20 μl; 3 mM) after 10, 45 and 120 min, and analysed by anion exchange HPLC (analytical Dionex DNAPac column) using the conditions as described above. Aminopurine fluorescence assays: cleavage kinetics Rate constants k obs for the U3AP–U54A variant were measured under pseudo-first-order conditions with Mg 2+ in excess over RNA. Stock solutions were prepared for the U3AP–U54A variant (concentration of each stran c RNA =0.5 μM in 50 mM KMOPS, pH 7.5, 100 mM KCl) and for MgCl 2 (concentration c MgCl2 =10 mM in 50 mM KMOPS; 100 mM KCl pH 7.5, 7.0 or 6.5 as indicated). Mixing of 120 μl RNA stock solution and of 1.2 μl MgCl 2 stock solution manually resulted in a final concentration of 0.5 μM RNA and 10 μM MgCl 2 . Spectra were recorded on a Varian Cary Eclipse spectrometer at 10, 15 or 20 °C using the following instrumental parameters: excitation wavelength, 308 nm; emission wavelength, 372 nm; increment of data point collection, 0.05 s; slit widths, 10 nm. The fluorescence data were fit to a single-exponential equation: F = A 1 + A 2 e −k′t ( A 1 : final fluorescence; A 2 e −k′t : change in fluorescence over time (t) at the observed rate k ′). The measurement for each concentration was repeated at least three times. The observed rate value provided is an arithmetic mean, determined from at least three independent stopped-flow measurements. All data processing was performed using Kaleidagraph software (Synergy Software). Accession codes : Protein Data Bank (PDB): The atomic coordinates and structure factors have been deposited under the following accession codes: 4RGE for dU5-containing env22 twister ribozyme, and 4RGF for same ribozyme crystals in Mn 2+ soaks. How to cite this article: Ren, A. et al. In-line alignment and Mg 2+ coordination at the cleavage site of the env22 twister ribozyme. Nat. Commun. 5:5534 doi: 10.1038/ncomms6534 (2014).